Conditional deletion ofMecp2in parvalbumin-expressing GABAergic cells results in the absence of critical period plasticity Mutations in the X-linked gene encoding the transcriptional modulator methyl–CpG-binding protein 2 (MeCP2) impair postnatal development of the brain. Here we use neuronal-type specific gene deletion in mice to show that conditional Mecp2 deletion in GABAergic parvalbumin-expressing (PV) cells ( PV-Mecp2 −/y ) does not cause most Rett-syndrome-like behaviours, but completely abolishes experience-dependent critical period plasticity of primary visual cortex (V1) that develops normal visual functions. However, selective loss of Mecp2 in GABAergic somatostatin-expressing cells or glutamatergic pyramidal cells does not affect the critical period plasticity. MeCP2-deficient PV cells exhibit high intrinsic excitability, selectively reduced efficacy of recurrent excitatory synapses in V1 layer 4 circuits, and decreased evoked visual responses in vivo . Enhancing cortical gamma-aminobutyric acid (GABA) inhibition with diazepam infusion can restore critical period plasticity in both young and adult PV-Mecp2 −/y mice. Thus, MeCP2 expression in inhibitory PV cells during the critical period is essential for local circuit functions underlying experience-dependent cortical plasticity. Rett syndrome (RTT) is a neurodevelopmental disorder majorly caused by loss-of-function mutations in the X-linked gene encoding the transcriptional modulator methyl−CpG-binding protein 2 (MeCP2) [1] , [2] . Typical RTT primarily affects girls and is characterized by a brief period of apparently normal development followed by the emergence of the loss of language, cognitive deficits, autistic features, motor abnormality and other neurological symptoms [2] , [3] . Mice lacking functional MeCP2 ( null , Mecp2 −/y ) recapitulate major features of RTT [4] , [5] . Both RTT patients and Mecp2 - null mice exhibit normal gross brain cytoarchitecture without detectable neuronal loss, implicating that changes in neural circuit functions are likely to be the cause of RTT phenotypes [4] , [6] , [7] . Indeed, Mecp2-null mice showed abnormality in neuronal dendrite morphology [6] , and dysfunction in synaptic circuits, including the reduction in synaptic efficacy and long-term potentiation (LTP) at excitatory synapses [8] , [9] , [10] , alteration in excitation–inhibition balance [8] , [11] , as well as defects in cortical inhibitory GABAergic connectivity and regression of visual function [12] . However, the use of germline Mecp2 -null mice may mask the direct consequence of MeCP2 dysfunction in neural circuits [2] , [13] . Specific deletion of Mecp2 in different neuronal types in various brain areas may contribute to the deficit of a particular behavioural phenotype [14] , [15] , [16] , [17] . In particular, selective Mecp2 deletion in GABAergic neurons reproduces most behavioural defects found in Mecp2-null mice [18] , suggesting MeCP2 deficiency in GABAergic neurons plays a critical role in RTT. The MeCP2-deficient GABAergic neurons show substantial reduction in gamma-aminobutyric acid (GABA) synthesis and inhibitory synaptic transmission, without significant change in excitatory synapses [18] . It remains unclear how specific GABAergic synaptic defects alter neural circuit development and plasticity, which may underlie Mecp2 mutation-induced behavioural phenotypes. Development of functional neural circuits requires synaptic refinements by sensory experience during a defined postnatal time window known as the critical period. It is best exemplified by visual experience-induced ocular dominance (OD) plasticity of the developing primary visual cortex (V1), in which monocular visual deprivation (MD) of one eye during the postnatal critical period results in a permanent loss of cortical neuronal responses to the deprived eye and a shift of OD towards the non-deprived eye [19] , [20] , [21] , [22] , [23] . Previous studies have shown that parvalbumin (PV)-expressing fast-spiking cells, a major type of GABAergic interneurons in the cortex, play a key role in regulating the onset of critical period for OD plasticity [22] , [24] , [25] . In the present study, using conditional knockout (KO) of Mecp2 in these inhibitory PV cells, we find that the critical period for OD plasticity is completely absent in the mouse V1, while the normal visual cortical functions are intact. Two-photon imaging guided recording shows that MeCP2-deficient cortical PV cells display significant decreased visually evoked spike response but relatively normal visual functional selectivity. Consistently, extensive paired recordings of layer 4 local circuits reveal that the basal efficacy of excitatory synaptic transmission from the pyramidal cell (PC) to PV cell is selectively decreased in mice with conditional deletion of Mecp2 in PV cells, resulting in reduced recurrent inhibition in the local cortical circuit. Furthermore, enhancing GABA inhibition with cortical infusion of benzodiazepam fully restores the normal OD plasticity. These results suggest that MeCP2-dependent local cortical circuit function is critical for regulating experience-dependent cortical plasticity during early postnatal development. PV-Mecp2 −/y mice do not show most RTT-like behaviours To delete Mecp2 in specific neuronal types, we generated conditional deletion of Mecp2 by crossing flox-Mecp2 female mice ( Mecp2 tm1Bird ) [5] with different Cre lines (males) that express Cre recombinase (Cre) in different neuronal types [26] . Only the male littermates were used for all following studies. In the first set of experiments, we selectively deleted Mecp2 from PV-positive fast-spiking cells by crossing Mecp2 tm1Bird with PV-Cre mice. To confirm the efficacy of conditional Mecp2 KO, we conducted immunostaining to compare the MeCP2 expression in the mouse V1 between the conditional KO mice PV-Cre;Mecp2 tm1Bird ( PV-mecp2 −/y ) and littermate controls, including wild-type (WT), PV-Cre and flox-Mecp2 alleles. In these control mice, we found that MeCP2 protein was expressed in all layers of V1 neurons in mice at postnatal day 30 (P30) and strong immunoreactivity was localized to the nuclei ( Fig. 1a (top) and Fig. 1b from PV-Cre mice). The expression of Cre in PV-Cre mice starts at P12 and reaches adequate level around P30 (refs 26 , 27 . Thus, in the PV-Mecp2 −/y mice MeCP2 expression decreased gradually in cortical PV cells starting around P20, and at P30 and P60 MeCP2 was absent in most GABAergic PV cells in the V1 (percentage of MeCP2-positive cells, P20: 85.4±2.0%, n =5 mice; P30: 17.8±2.6%, n =7 mice; P60: 13.9±1.2%, n =3 mice, Fig. 1a (bottom) and Fig. 1b ). In contrast, MeCP2 remained high expression level in glutamatergic excitatory PCs and other neuronal types in PV-Mecp2 −/y mice ( Fig. 1a bottom). Moreover, the density of PV cell in the developing V1 remained unchanged in the comparison between different alleles ( Fig. 1b , bottom), suggesting there is no loss of cortical PV cells. These results confirmed the efficacy of conditional Mecp2 deletion in PV cells of mice around P30, a peak time for experience-dependent mouse V1 circuit plasticity [21] . 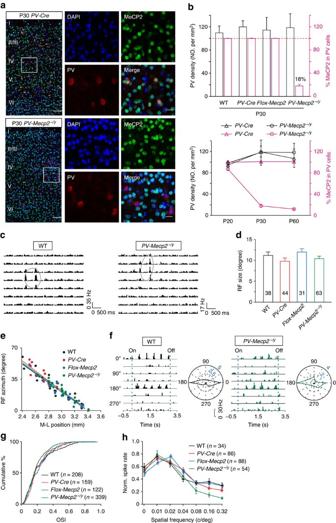Figure 1: Normal visual cortical functions inPV-Mecp2−/ymice. (a) Fluorescence images showing V1 sections stained for the nucleus (4′,6-diamidino-2-phenylindole, DAPI), MeCP2 and parvalbumin (PV). Right: higher resolution images of the rectangle area. Scale bars, 100 and 20 μm for low and high resolution images, respectively. (b) Plots of the density of PV cells (black) and the percentage of MeCP2-immunostaining cells in total PV cells (magenta) in the V1 of different types of mice at P30 (upper) and over the postnatal development (P20–60) inPV-CreandPV-Mecp2−/ymice (bottom). (c) Contralateral RFs of example V1 binocular cells recorded in the WT andPV-Mecp2−/ymice at P30. Peri-stimulation histograms (PSTHs) of spike rate in response to flashing bright square (about 10°) at discrete positions in an 8 × 8 grid were shown. Red lines outline the approximate size of the RFs. (d) The mean RF size of V1 binocular cells recorded in WT (black),PV-Cre(red),flox-Mecp2(blue) andPV-Mecp2−/y(green) mice. (e) Plot of V1 cell RF-centre azimuths relative to the vertical meridian (M–L position) from WT,PV-Cre,flox-Mecp2andPV-Mecp2−/ymice. (f) PSTH and polar plots of spike rates evoked by drifting gratings at eight different orientations (45° step; spatial frequency 0.002 cycle per degree; temporal frequency 2 Hz) of example V1 cells recorded from WT (black) andPV-Mecp2−/y(red) mice. Blue dashed lines: stimulation duration. The numbers in blue represent spike rates. (g) Cumulative percentage distribution of orientation selectivity indices (OSIs) for all recorded V1 cells from WT,PV-Cre,flox-Mecp2andPV-Mecp2−/ymice. No significant difference was found between the data from paired genotypes (Kolmogorov–Smirnov test). (h) The dependence of spike rate on the spatial frequency of drifting gratings of V1 cells from four genotypes. Average data are presented as mean±s.e.m. Figure 1: Normal visual cortical functions in PV-Mecp2 −/y mice. ( a ) Fluorescence images showing V1 sections stained for the nucleus (4′,6-diamidino-2-phenylindole, DAPI), MeCP2 and parvalbumin (PV). Right: higher resolution images of the rectangle area. Scale bars, 100 and 20 μm for low and high resolution images, respectively. ( b ) Plots of the density of PV cells (black) and the percentage of MeCP2-immunostaining cells in total PV cells (magenta) in the V1 of different types of mice at P30 (upper) and over the postnatal development (P20–60) in PV-Cre and PV-Mecp2 −/y mice (bottom). ( c ) Contralateral RFs of example V1 binocular cells recorded in the WT and PV-Mecp2 −/y mice at P30. Peri-stimulation histograms (PSTHs) of spike rate in response to flashing bright square (about 10°) at discrete positions in an 8 × 8 grid were shown. Red lines outline the approximate size of the RFs. ( d ) The mean RF size of V1 binocular cells recorded in WT (black), PV-Cre (red), flox-Mecp2 (blue) and PV-Mecp2 −/y (green) mice. ( e ) Plot of V1 cell RF-centre azimuths relative to the vertical meridian (M–L position) from WT, PV-Cre , flox-Mecp2 and PV-Mecp2 −/y mice. ( f ) PSTH and polar plots of spike rates evoked by drifting gratings at eight different orientations (45° step; spatial frequency 0.002 cycle per degree; temporal frequency 2 Hz) of example V1 cells recorded from WT (black) and PV-Mecp2 −/y (red) mice. Blue dashed lines: stimulation duration. The numbers in blue represent spike rates. ( g ) Cumulative percentage distribution of orientation selectivity indices (OSIs) for all recorded V1 cells from WT, PV-Cre , flox-Mecp2 and PV-Mecp2 −/y mice. No significant difference was found between the data from paired genotypes (Kolmogorov–Smirnov test). ( h ) The dependence of spike rate on the spatial frequency of drifting gratings of V1 cells from four genotypes. Average data are presented as mean±s.e.m. Full size image Previous study has shown that mice with MeCP2 deficiency in all GABAergic neurons recapitulate RTT-like behaviours [18] . In the present study, we found that the PV-Mecp2 −/y and control mice (WT, PV-Cre and flox-Mecp2 ) littermates were generally healthy and did not exhibit most of apparent RTT-like behavioural phenotype as they reached adulthood. In the behavioural tests on 8- to 10-week-old mice, our results showed that the PV-Mecp2 −/y mice exhibited apparent defects in motor coordination and motor learning, with shorter latency to fall on the accelerating rotarod at 8 weeks in comparison with that of WT, PV-Cre and flox-Mecp2 control mice ( Supplementary Fig. 1a ), while the locomotion remained normal as reflected by the normal travel distance within a 30-min period in the open-field test ( Supplementary Fig. 1e ). However, we did not find any defects of social interaction in the three-chamber test ( Supplementary Fig. 1b ) and apparent anxiety-like phenotypes in the elevated plus maze, light–dark box and open-field test (the centre distance) in PV-Mecp2 −/y mice at 10 weeks ( Supplementary Fig. 1c–e ). Furthermore, in the contextual/cue memory test, PV-Mecp2 −/y mice displayed trends towards shorter freezing time, suggesting a potential impairment of fear memory ( Supplementary Fig. 1f ). Overall, these behavioural test results suggest that conditional deletion of Mecp2 from PV cells at early postnatal period does not result in apparent RTT-like behaviours, except for motor dysfunctions. PV-Mecp2 −/y mice exhibit normal visual cortical functions We next tested whether the specific deletion of Mecp2 from GABAergic PV cells impairs cortical sensory processing functions by assessing visual function properties of developing V1. We used glass micropipette to extracellularly record single-unit spiking activities in the binocular zone of mouse V1 at P28–30, under the anaesthesia with ketamine/medetomidine. The receptive fields (RFs) of cortical neurons (mapped with 8 × 8 grids of spare-noise stimuli, see Methods) exhibited similar size and spatial structure in both WT and PV-Mecp2 −/y mice ( Fig. 1c ), and the mean size of RFs did not show significant difference among WT, PV-Cre , flox-Mecp2 and PV-Mecp2 −/y mice ( Fig. 1d ). We also assessed the retinotopic organization by plotting RF-centre azimuth versus microelectrode recording positions relative to vertical meridian medial to lateral axis (M−L), and found no significant difference among the four different genotypes of littermates ( Fig. 1e ). Moreover, the orientation selectivity of individual neurons was examined by measuring neuronal spiking rates in response to drifting gratings with eight different orientations, as shown in the example cell from a WT or a PV-Mecp2 −/y juvenile mouse in Fig. 1f . Using the global orientation selectivity index (OSI, see Methods), we quantified the orientation selectivity for all recorded V1 cells and found that OSI distributions were not significantly different among WT, PV-Cre , flox-Mecp2 and PV-Mecp2 −/y mice around P28–30 ( Fig. 1g ). Further measurements of spatial frequency dependence of neuronal response also showed similar preference for low spatial frequency stimuli in the controls and PV-Mecp2 −/y juvenile mice ( Fig. 1h ). Thus, all these visual physiology results indicate that conditional deletion of Mecp2 in PV cells during the critical period does not result in obvious defects in the development of visual functions of cortical neurons. This is consistent with the recent finding that postnatal Mecp2 -deletion in PV cells did not impair visual cortical functions, for example, visual acuity function, in the juvenile mice, while severe regression of visual function was observed in Mecp2-null mice [12] . Absence of critical period plasticity in PV-Mecp2 −/y mice Given that normal visual cortical functions were intact in PV-Mecp2 −/y mice, we further examined the effect of conditional Mecp2 deletion in PV cells on visual experience-dependent OD plasticity of the V1 during the critical period. To assay the critical period plasticity of mouse V1, the effect of 4-d MD (beginning at P26, see Methods) on the OD preference of neuronal spike responses in the V1 binocular zone was examined at the end of deprivation in vivo [21] . In WT mice, 4-d MD of the contralateral eye input with eyelid suture resulted in an apparent shift of cortical neuronal responses from the contralateral eye towards the ipsilateral eye, as assayed by the OD index (ODI), which represents the normalized difference between responses elicited by inputs from the two eyes [21] . This effect of MD could also be depicted by the classical 7-scale histogram of OD by grouping ODIs into seven categories [23] ( Fig. 2a , top two panels), and the ocular preference bias of all 7-group neurons can then be summarized by a single contralateral bias index (CBI) [21] . The distributions of ODIs as shown by the cumulative percentage plots for all neurons showed marked difference between the normal-reared and MD-treated groups of WT mice ( P =5.5 × 10 −6 , Kolmogorov–Smirnov test; Fig. 2a , bottom panel). In contrast to WT mice, we found that same MD treatment in PV-Mecp2 −/y mice during P26-30 did not induce any significant shift in the OD distribution, exhibiting little difference in the CBI values and ODI distributions ( Fig. 2b ; P =0.93, Kolmogorov–Smirnov test). As controls, we found similar OD shifts in 4-d MD PV-Cre and flox-Mecp2 littermates as that found in WT mice ( Fig. 2c,d ), although the flox-Mecp2 alleles exhibited a reduced level of MeCP2 protein in the brain [28] . By contrast, we found that 4-d MD during the critical period in mice with conditional deletion in somatostatin-expressing (Sst) GABAergic cells ( Sst-Cre; Mecp2 tm1Bird littermates, Sst-Mecp2 −/y ; Supplementary Fig. 2a ), another major subtype of inhibitory interneurons, still effectively caused similar OD shifts of the V1 as that found in WT mice ( Fig. 2e ), so did the mice lacking Mecp2 selectively from glutamatergic excitatory PCs (Nex-Cre; Mecp2 tm1Bird littermates, Nex-Mecp2 −/y ; Fig. 2f and Supplementary Fig. 2b ). Thus, these results suggest that specific deletion of Mecp2 in PV cell circuits causes the absence of critical period plasticity. 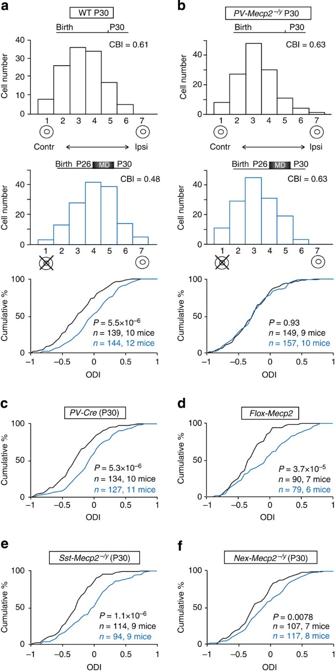Figure 2: OD plasticity in wild type and mice with specificMecp2deletion in different neuronal types. (a) Top: 7-Scale histograms of OD of V1 neurons based on the measured OD index (ODI) from normally reared (black) and 4-d MD (blue) young WT mice, with calculated CBI. ‘Contra’ and ‘Ipsi’ refer to preferential responses to inputs from the contra- and ipsilateral eyes, respectively, and the cross represents the visual deprivation. Bottom: Cumulative percentage distribution of ODI shown in top. ODI ranges from +1 for neurons driven exclusively by the ipsilateral eye to −1 for those driven exclusively by the contralateral eye. (b) 7-Scale histograms and cumulative percentage distribution of ODIs for youngPV-Mecp2−/ymice with (blue) and without (black) MD treatment. (c–f) Cumulative percentage distributions for ODIs with (blue) and without (black) MD treatment. Data collected from: (e) P30PV-Creand P30flox-Mecp2, (f) P30Sst-Mecp2−/yand (g) P30Nex-Mecp2−/y.P-values were calculated by Kolmogorov–Smirnov test. Figure 2: OD plasticity in wild type and mice with specific Mecp2 deletion in different neuronal types. ( a ) Top: 7-Scale histograms of OD of V1 neurons based on the measured OD index (ODI) from normally reared (black) and 4-d MD (blue) young WT mice, with calculated CBI. ‘Contra’ and ‘Ipsi’ refer to preferential responses to inputs from the contra- and ipsilateral eyes, respectively, and the cross represents the visual deprivation. Bottom: Cumulative percentage distribution of ODI shown in top. ODI ranges from +1 for neurons driven exclusively by the ipsilateral eye to −1 for those driven exclusively by the contralateral eye. ( b ) 7-Scale histograms and cumulative percentage distribution of ODIs for young PV-Mecp2 −/y mice with (blue) and without (black) MD treatment. ( c – f ) Cumulative percentage distributions for ODIs with (blue) and without (black) MD treatment. Data collected from: ( e ) P30 PV-Cre and P30 flox-Mecp2 , ( f ) P30 Sst-Mecp2 −/y and ( g ) P30 Nex-Mecp2 −/y . P -values were calculated by Kolmogorov–Smirnov test. Full size image We further examined whether the absence of MD-induced OD plasticity during the early postnatal period is due to the delay of critical period onset. In the tests of visual properties of V1 cells in adult mice during the period of P60–120, we again found that the RFs size and azimuth of recorded adult V1 cells showed no significant difference between WT and PV-Mecp2 −/y mice ( Fig. 3a,b ). Compared with adult WT mice, adult PV-Mecp2 −/y mice showed normal orientation selectivity, quantified by OSI ( Fig. 3c ), and spatial frequency selectivity ( Fig. 3d ). These results indicate that the V1 of adult PV-Mecp2 −/y mice possesses normal visual functions. Furthermore, there was no significant difference in visual functional properties of V1 cells between the juvenile (P28–30) and adult stages in both WT and PV-Mecp2 −/y mice ( Fig. 3a–d versus Fig. 1d–h ), further suggesting that the expression of MeCP2 in PV cells is not required for the development and maintenance of general visual functions of the V1 during the postnatal period. Similar finding was reported by a recent study reporting that visual acuity were normal in adult PV-Mecp2 −/y mice but severely impaired in Mecp2-null mice [12] . Interestingly, we again found that in the adult PV-Mecp2 −/y mice, there was still no significant OD shift following the 4-d MD treatment ( Fig. 3f ), while similar 4-d MD caused a smaller but significant OD shift in the adult WT mice ( Fig. 3e ) in comparison with that observed during the critical period ( Fig. 1a ). Taken together, the results from mice in both the critical period and adult suggest that selective postnatal Mecp2 deletion in PV cells results in an absence of experience-dependent OD plasticity in the V1. 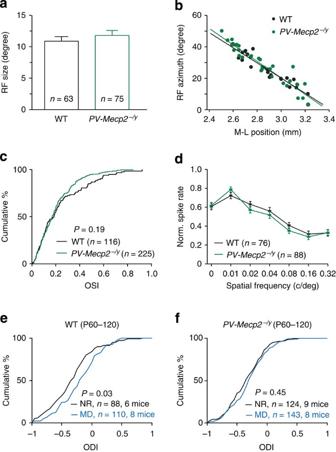Figure 3: Intact V1 function and aberrant OD plasticity in adultPV-Mecp2−/ymice. (a) The mean RF size of V1 binocular cells recorded in adult WT (black) andPV-Mecp2−/y(green) mice (P=0.35,t-test). (b) Plot of V1 cells RF-centre azimuths relative to the M−L position from adult WT andPV-Mecp2−/ymice. (c) Cumulative percentage distribution of orientation selectivity indices (OSIs) from all V1 cells from adult WT andPV-Mecp2−/ymice. No significance was found between the data from the two genotypes (P=0.19, Kolmogorov–Smirnov test). (d) The dependence of spike rate on the spatial frequency of drifting gratings of all recorded V1 cells from adultWTandPV-Mecp2−/ymice. (e,f) Cumulative percentage distributions of ODIs for all recorded cells with (blue) and without (black) MD treatment from adult WT (e) andPV-Mecp2−/y(f) mice.P-values were calculated by the Kolmogorov–Smirnov test. Average data are presented as mean±s.e.m. Figure 3: Intact V1 function and aberrant OD plasticity in adult PV-Mecp2 −/y mice. ( a ) The mean RF size of V1 binocular cells recorded in adult WT (black) and PV-Mecp2 −/y (green) mice ( P =0.35, t -test). ( b ) Plot of V1 cells RF-centre azimuths relative to the M−L position from adult WT and PV-Mecp2 −/y mice. ( c ) Cumulative percentage distribution of orientation selectivity indices (OSIs) from all V1 cells from adult WT and PV-Mecp2 −/y mice. No significance was found between the data from the two genotypes ( P =0.19, Kolmogorov–Smirnov test). ( d ) The dependence of spike rate on the spatial frequency of drifting gratings of all recorded V1 cells from adult WT and PV-Mecp2 −/y mice. ( e , f ) Cumulative percentage distributions of ODIs for all recorded cells with (blue) and without (black) MD treatment from adult WT ( e ) and PV-Mecp2 −/y ( f ) mice. P -values were calculated by the Kolmogorov–Smirnov test. Average data are presented as mean±s.e.m. Full size image Visual functions of MeCP2-deficient cortical PV cells As cortical PV cells constitute 8–10% of all neurons in the mouse cortex and distribute unevenly across cortical six layers [29] . The majority of visual cortical neurons we recorded in vivo were excitatory PCs. To directly examine whether the specific deletion of Mecp2 in PV cells would affect their neuronal functions, we performed in vivo cell-attached recording from cortical PV cells in PV-Cre;Ai9 or PV-Mecp2 −/y ;Ai9 mice ( Fig. 4a ), in which the fluorescence protein tdTomato was specifically expressed in PV cells via crossing the reporter mice Ai9 (ref. 26 ) with PV-Cre or PV-Mecp2 −/y mice. Consistent with previous studies [30] , [31] , [32] , we found that the layer 2/3 PV cells recorded from both two genotypes in adult period (~P60) discharged narrower spikes at higher rate and had relative larger size of RFs, as well as broadened orientation tuning ( Fig. 4a–c ), in comparison with the visual response properties of V1 excitatory cells examined in previous extracellular recording experiments ( Figs 1c–g and 3a–c ). However, we found that the RF property and the orientation tuning of cortical PV cells were not significantly different between PV-Cre;Ai9 control and PV-Mecp2 −/y ;Ai9 KO mice ( Fig. 4b,c ; OSI of control PV cells: 0.17±0.027, n =26 from 7 mice; OSI of MeCP2-deficient PV cells: 0.12±0.028, n =19 from 4 mice; P =0.31, Kolmogorov–Smirnov test). We noted that in the orientation tuning test, the drifting grating-evoked average spiking rate (across the 12 orientations) of cortical PV cell was significantly lower in PV-Mecp2 −/y ;Ai9 mice than PV-Cre;Ai9 mice ( Fig. 4c,d , right panel, P =0.03, t -test), while average spontaneous spiking rate of these neurons remained at similar levels ( Fig. 4d , left panel, P =0.26). Moreover, similar to control mice, layer 2/3 PV cells in PV-Mecp2 −/y ;Ai9 mice still had their strong preferences for low spatial and temporal frequencies of visual stimuli, respectively, although these MeCP2-deficient cells showed overall weaker spiking responses to drifting gratings with varying spatial or temporal frequency, respectively ( Fig. 4e ). These results directly suggest that the Mecp2 deletion in cortical PV cells selectively decreases their visual input-induced spiking responses, but does not alter their general tuning properties to visual inputs. 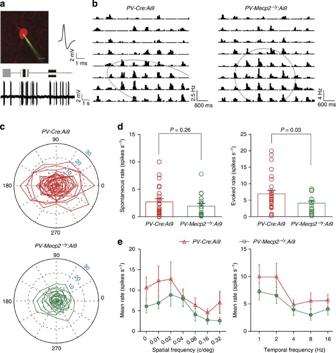Figure 4: Visual functions of cortical PV cells in adultPV-Cre;Ai9andPV-Mecp2−/y;Ai9mice. (a) Top: Two-photon laser imaging of a tdTomato-expressing cortical PV cell (red) and an example trace of extracellular spike. The recording micropipette was filled with Alex fluor-488 (green). Scale bar, 20 μm. Bottom: Spikes evoked by drifting gratings from the recorded PV cell. (b) Receptive fields of an example V1 PV cell recorded from adultPV-Cre;Ai9(left) andPV-Mecp2−/y;Ai9mice (right). (c) Polar plots of spike response preferences of all examined cortical PV cells in adultPV-Cre;Ai9(red,n=26 cells from 7 mice, top) andPV-Mecp2−/y;Ai9mice (green,n=19 cells from 4 mice, bottom). (d) The magnitudes of averaged baseline spontaneous (left) and evoked spike activity (right) of cortical PV cells from the experiments inc. Each dot represents data from a cell, and bars are mean±s.e.m. Thet-test was used. (e) The dependence of spike rate on the spatial (left) or temporal (right) frequency of drifting gratings at the optimal orientation of adult cortical PV cells. No significant difference was found between the two genotypes. Figure 4: Visual functions of cortical PV cells in adult PV-Cre;Ai9 and PV-Mecp2 −/y ;Ai9 mice. ( a ) Top: Two-photon laser imaging of a tdTomato-expressing cortical PV cell (red) and an example trace of extracellular spike. The recording micropipette was filled with Alex fluor-488 (green). Scale bar, 20 μm. Bottom: Spikes evoked by drifting gratings from the recorded PV cell. ( b ) Receptive fields of an example V1 PV cell recorded from adult PV-Cre;Ai9 (left) and PV-Mecp2 −/y ;Ai9 mice (right). ( c ) Polar plots of spike response preferences of all examined cortical PV cells in adult PV-Cre;Ai9 (red, n =26 cells from 7 mice, top) and PV-Mecp2 −/y ;Ai9 mice (green, n =19 cells from 4 mice, bottom). ( d ) The magnitudes of averaged baseline spontaneous (left) and evoked spike activity (right) of cortical PV cells from the experiments in c . Each dot represents data from a cell, and bars are mean±s.e.m. The t -test was used. ( e ) The dependence of spike rate on the spatial (left) or temporal (right) frequency of drifting gratings at the optimal orientation of adult cortical PV cells. No significant difference was found between the two genotypes. Full size image Altered membrane properties of PV cells in PV-Mecp2 −/y mice How does conditional Mecp2 deletion in PV cells affect neural circuit functions that underlie the critical period plasticity? We addressed this question by examining neuronal properties and synaptic functions of the V1 layer 4 local circuits in acute cortical slices from WT, flox-Mecp2 , PV-Cre;Ai9 and PV-Mecp2 −/y ;Ai9 mice at P28–30 or P50–55, using whole-cell recording. The V1 layer 4 is the main thalamorecipient lamina that transfers visual information into the cortex. In this sets of experiments, we specifically targeted PV cells in cortical slices by the expression of tdTomato in PV-Cre;Ai9 and PV-Mecp2 −/y ;Ai9 mice, while in the brain slices from WT or flox-Mecp2 mice, the cortical fast-spiking PV cells were initially identified by their rough morphology under the infrared camera and further confirmed by their intrinsic non-accommodating high-rate firing pattern and reconstructed morphology after the recording [33] , [34] , [35] . Excitatory PCs in the same layer were easily identified by their clear apical dendrites and low firing rates with adaptation. We first examined the passive membrane properties and the intrinsic excitability of the layer 4 PCs and PV cells, respectively, by intracellular injection of step currents (600 ms duration, current steps of 40–50 pA) in the current-clamp mode ( Fig. 5a,c ). Compared with those PV cells recorded in slices from the WT, flox-Mecp2 or PV-Cre;Ai9 control mice at ~P30, MeCP2-deficient PV cells exhibited higher membrane resistance ( P =0.01 versus WT, t -test) and lower current threshold (rheobase, P =0.002) for generating the action potential, as well as relatively more hyperpolarized membrane potential threshold for action potentials ( P =0.03) ( Table 1 and Fig. 5b ). These intrinsic properties are reminiscent to functional characteristics of immature PV cells [36] . By contrast, no significant difference was found in most membrane properties of layer 4 PCs recorded in the same slices between controls and PV-Mecp2 −/y ;Ai9 mice ( Table 1 and Fig. 5c,d ). By measuring whole-cell currents of K + and Na + channels and their voltage dependence in layer 4 PV cells with specified stepped-voltage clamping protocols, respectively, we found a reduction of the density of both K + and Na + channels in the membrane and a shift of the half activation voltage ( V 1/2 ) of overall K + currents in these MeCP2-deficient PV cells at ~P30 in comparison with these from PV-Cre;Ai9 control mice ( Supplementary Fig. 3 ). These changes of major membrane channels in MeCP2-deficient PV cells could partially account for their relatively immature membrane functions. At P50, these MeCP2-deficient PV cells also exhibited much higher membrane resistance ( P =0.034, t -test) and smaller membrane capacitance ( P =0.008), compared with that at P30 ( Table 1 ). The slope of I / O curve (neuronal gain) was significantly steeper in adult MeCP2-deficient PV cells than that at P30 ( Table 1 and Fig. 5e,f ). Thus, conditional Mecp2 deletion in PV cells during the postnatal critical period and adulthood selectively impaired the maturation of membrane functions of these cortical PV cells. 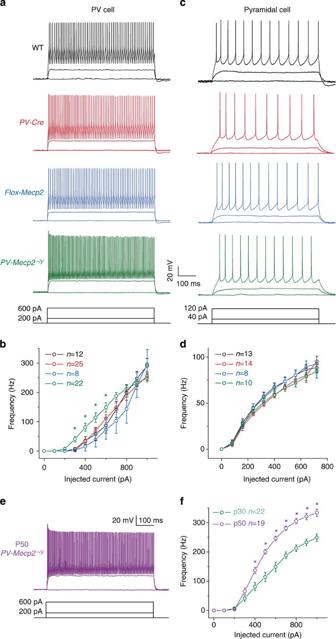Figure 5: Intrinsic excitability of layer 4 PV and PCs in the four different genotypes. (a) Example recording traces depicting action potential firing of PV cells in response to step depolarizing currents (duration 600 ms) in slices from P30 WT (black),PV-Cre(red),flox-Mecp2(blue) andPV-Mecp2−/y(green) mice. (b) Plot of evoked spike rates versus current magnitudes (I/Ocurve) of PV cells from WT and other three genotypes. *0.01<P<0.05,t-test. (c,d) Same tests on PC cells recorded from same slices of the four different genotypes. (e,f) Same tests on PV cells recorded from cortical slices of P50PV-Mecp2−/y(purple) mice.P-values were calculated byt-test when comparing with the data from P30PV-Mecp2−/y(light green). Average data are presented as mean±s.e.m. Figure 5: Intrinsic excitability of layer 4 PV and PCs in the four different genotypes. ( a ) Example recording traces depicting action potential firing of PV cells in response to step depolarizing currents (duration 600 ms) in slices from P30 WT (black), PV-Cre (red), flox-Mecp2 (blue) and PV-Mecp2 −/y (green) mice. ( b ) Plot of evoked spike rates versus current magnitudes ( I / O curve) of PV cells from WT and other three genotypes. *0.01< P <0.05, t -test. ( c , d ) Same tests on PC cells recorded from same slices of the four different genotypes. ( e , f ) Same tests on PV cells recorded from cortical slices of P50 PV-Mecp2 −/y (purple) mice. P -values were calculated by t -test when comparing with the data from P30 PV-Mecp2 −/y (light green). Average data are presented as mean±s.e.m. Full size image Table 1 Membrane properties of layer 4 PV and PCs from four mouse lines at different postnatal days. Full size table Synaptic dysfunction of cortical MeCP2-deficient PV cells We further examined the synaptic transmission in cortical PV cell circuits following the specific Mecp2 deletion in PV cells, by conducting extensive paired whole-cell recording from the layer 4 PV and PCs in visual cortical slices prepared from four different genotypes at P28–30. First, we found that the monosynaptic inhibitory postsynaptic currents (IPSCs) elicited in the PC by stimulating a neighbouring PV cell showed little difference in the amplitude between WT and PV-Cre , flox-Mecp2 , or PV-Mecp2 −/y mice ( P =0.70, 0.83 and 0.76 for PV-Cre , flox-Mecp2 and PV-Mecp2 −/y versus WT, respectively, t -test; Fig. 6a,b ). Tests using repetitive stimulation to the presynaptic PV cell at 20 Hz showed no significant difference in the short-term synaptic depression ( Fig. 6b , right). Moreover, after the five repetitive stimulation, the depressed GABAergic transmission from PV cells to neighbouring PCs showed a similar recovery level in all four genotypes ( P =0.14, 0.34 and 0.52 for PV-Cre , flox-Mecp2 and PV-Mecp2 −/y versus WT, respectively; Fig. 6b , right panel). These results suggested that the Mecp2 deletion in the cortical PV cell does not alter the normal function and short-term plasticity of its inhibitory output synapses onto excitatory PCs in the V1 layer 4. As major cortical PV cell population, for example, basket cells, are known to make perisomatic inhibitory synapses on neighbouring PCs [37] , we further conducted morphological assay of the density of PV axon terminals (labelled with tdTomato) surrounding the PC soma in cortical sections of PV-Cre;Ai9 control and PV-Mecp2 −/y ;Ai9 mice ( Supplementary Fig. 5a , see Methods). Using this morphological assay, we verified a time course of gradual increase in the density of PV axon terminals on the PC soma in the layers 2/3 and 4 of V1 during the critical period ( Supplementary Fig. 5b and see ref. 38 ), and further showed that at P30 and 60, the cortical PV puncta density was not significantly different between PV-Cre;Ai9 control and PV-Mecp2 −/y ;Ai9 mice ( Supplementary Fig. 5b ). This result is consistent with the recent study that showed unaffected density of immunohistochemically labelled perisomatic PV-positive puncta on cortical layer 4 PCs in mice with conditional loss of Mecp2 in these PV cells [12] . Thus, both electrophysiology and morphology results suggest that selective postnatal Mecp2 deletion in cortical PV cells does not alter the connectivity and function of PV cell inhibitory synapse onto the cortical excitatory PC cells. 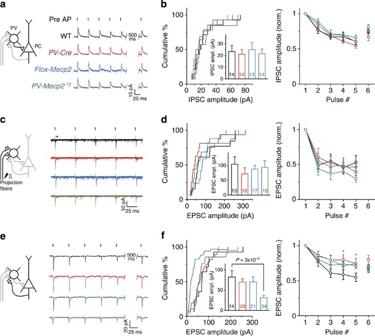Figure 6: Selective synaptic dysfunction of cortical layer-4 PV cells inPV-Mecp2−/ymice. (a) Diagram depicting the configuration for recording monosynaptic IPSCs in a PC (Vclamp=−40 mV) in response to electric stimulation to a neighbouring PV cell in acute V1 slices. Traces: sample IPSCs recorded from postsynaptic PCs in WT,PV-Cre(;Ai9),flox-Mecp2andPV-Mecp2−/y(;Ai9)mice, elicited by five consecutive PV cell action potentials (APs) at 20 Hz, followed by a single spike after 0.5 s. Scale bar, 10 pA, 25 ms. (b) Left: Cumulative distribution and the mean value (inset) of amplitudes of the first IPSC evoked by a train stimulation of all recorded pairs; Right: Short-term depression and synaptic recovery rate of recurrent inhibitory PV–PC synapses from the experiments shown ina.n, number of examined cells. (c,d) Diagram depicting the configuration for recording monosynaptic EPSCs in a PV cell (Vclamp=−70 mV) in response to electric stimulation of projection axons in the white matter region below layer 6. Scale bar, 50 pA, 25 ms. The asterisk indicates occasional transmission failure during the minimal stimulation. Data depicted in the same manner as ina,b. (e,f) Diagram depicting the configuration for the recording of monosynaptic EPSCs in a PV cell (Vclamp=−70 mV) in response to stimulation of a neighbouring PC. Scale bar, 20 pA, 25 ms. The EPSC amplitudes fromPV-Mecp2−/y(;Ai9)mice showed significant reduction in comparison with WT, (P=0.0003,t-test), but not at the same synapse fromPV-Cre(;Ai9)andflox-Mecp2mice (P=0.43 and 0.57, respectively). Average data are presented as mean±s.e.m. Figure 6: Selective synaptic dysfunction of cortical layer-4 PV cells in PV-Mecp2 −/y mice. ( a ) Diagram depicting the configuration for recording monosynaptic IPSCs in a PC ( V clamp =−40 mV) in response to electric stimulation to a neighbouring PV cell in acute V1 slices. Traces: sample IPSCs recorded from postsynaptic PCs in WT, PV-Cre(;Ai9) , flox-Mecp2 and PV-Mecp2 −/y (;Ai9) mice, elicited by five consecutive PV cell action potentials (APs) at 20 Hz, followed by a single spike after 0.5 s. Scale bar, 10 pA, 25 ms. ( b ) Left: Cumulative distribution and the mean value (inset) of amplitudes of the first IPSC evoked by a train stimulation of all recorded pairs; Right: Short-term depression and synaptic recovery rate of recurrent inhibitory PV–PC synapses from the experiments shown in a . n , number of examined cells. ( c , d ) Diagram depicting the configuration for recording monosynaptic EPSCs in a PV cell ( V clamp =−70 mV) in response to electric stimulation of projection axons in the white matter region below layer 6. Scale bar, 50 pA, 25 ms. The asterisk indicates occasional transmission failure during the minimal stimulation. Data depicted in the same manner as in a , b . ( e , f ) Diagram depicting the configuration for the recording of monosynaptic EPSCs in a PV cell ( V clamp =−70 mV) in response to stimulation of a neighbouring PC. Scale bar, 20 pA, 25 ms. The EPSC amplitudes from PV-Mecp2 −/y (;Ai9) mice showed significant reduction in comparison with WT, ( P =0.0003, t -test), but not at the same synapse from PV-Cre(;Ai9) and flox-Mecp2 mice ( P =0.43 and 0.57, respectively). Average data are presented as mean±s.e.m. Full size image Second, excitatory inputs from distant neurons to cortical layer 4 PV cells, primarily from thalamocortical projection neurons [39] , were also examined by recording monosynaptic excitatory postsynaptic currents (EPSCs) elicited by minimal electric stimulation in the white matter below layer 6. The GABA A receptor antagonist picrotoxin (PTX, 20 μM) was used to block the evoked feed-forward inhibitory transmission in this set of experiments. Again, we found that the EPSC amplitude and short-term plasticity of these projection excitatory synapses were not significantly different between PV-Mecp2 −/y and three different control genotypes (WT, PV-Cre or flox-Mecp2 ; Fig. 6c,d ), suggesting unaffected thalamocortical excitatory inputs following the Mecp2 deletion in PV cells. We also checked these projection synapses on layer 4 excitatory PCs in the absence of PTX. Our results suggest that both the EPSC amplitude and short-term plasticity of these synapses, tested by minimal intensity of electric stimuli to the axonal fibres, do not show significant change among the four genotypes ( Supplementary Fig. 4a,b ). By increasing the intensity of electric stimuli to the projection fibres, we further demonstrated that the ratio of excitatory and inhibitory conductances in cortical layer 4 PCs retained the similar values among all four genotypes ( Supplementary Fig. 4c–e ), suggesting an unchanged excitation/inhibition balance in the thalamocortical feed-forward inputs. Taken together, these data suggest that the inhibitory ‘gating’ function of cortical layer 4 PV cells on thalamocortical inputs is not altered in PV-Mecp2 −/y mice. Finally, we found that in the layer 4 PV cells of PV-Mecp2 −/y mice, the strength of recurrent excitatory inputs from a neighbouring PC reduced to half of that found in WT mice ( P =0.0003; Fig. 6e,f ), while recording from PV-Cre or flox-Mecp2 mouse slices did not show a significant change in the strength at same synapses ( P =0.43 and 0.57 for PV-Cre and flox-Mecp2 versus WT, respectively; Fig. 6e,f ). However, the rates of short-term depression and synaptic recovery at these local recurrent excitatory synapses in flox-Mecp2 and PV-Mecp2 −/y mice were not significantly different from that found in WT mice, except that slightly less depression was found for the fourth ( P =0.04, versus WT, t -test) and fifth ( P =0.01) stimuli in PV-Cre mice ( Fig. 6f , right). This result implied a postsynaptic change of the recurrent excitatory synapse on MeCP2-deficient layer 4 PV cells. In contrast, at recurrent PC–PC synapses within the same layer, there was no significant difference in the connection probability (<10%), as well as the mean unitary synaptic strength and short-term depression between PV-Mecp2 −/y and WT mice at P30 ( Supplementary Fig. 4f–h ). Taken together, the above electrophysiology analysis of cortical synapses in the layer 4 circuits directly suggests that the conditional deletion of Mecp2 in PV cells has resulted in selective deficiency in their excitatory inputs within the layer 4 local circuit, without affecting their local inhibitory output and major excitatory input from the thalamus. Besides, such PV cell-specific Mecp2 deletion also did not affect thalamocortical feed-forward inputs to cortical PCs and recurrent cortical PC–PC synapses in the layer 4. Altered transcription of major genes in PV-Mecp2 −/y mice To reveal molecular basis for the altered neuronal/synaptic dysfunctions in PV-Mecp2 −/y mice, we performed quantitative reverse transcriptase–PCR (qRT–PCR) to measure the transcription changes of related functional genes. Using fluorescence-activated cell sorting (FACS), we harvested genetically tdTomato-labelled PV cells from the V1 of PV-Cre;Ai9 or PV-Mecp2 −/y ;Ai9 mice (P30) and non-fluorescent cortical cells, which served as internal control for each batch of qRT–PCR experiments ( Supplementary Fig. 5c , see Methods). In the samples from PV-Mecp2 −/y ;Ai9 mice, a reduced MeCP2 expression by ~60% specifically in tdTomato-positive PV cell groups, instead of non-fluorescence cells (values were normalized to that from PV-Cre;Ai9 control mice, Table 2 ), indicated a practically good sorting efficiency with the FACS. As shown by qRT–PCR results for five categories of functional genes in Table 2 , the tdTomato-labelling MeCP2-deficient cortical PV cells showed considerable reduction of relative messenger RNA levels of genes, including Parvalbumin , Gad2 , Calretinin (GABA function), Kv3.1 (a PV cell-enriched K + ionic channel), Gabra1 , Gabra2 (GABA A receptor α subunits) and Glur3 (a glutamate receptor subunit GluR3). The transcription reduction of these genes could account for alterations in neuronal/synaptic functions in MeCP2-deficient PV cells to some degree. For example, reduced expression of Kv3.1 and Glur3 correlated well with the higher input resistance ( Table 1 and Fig. 5a,b ) and the reduced recurrent excitatory inputs ( Fig. 6f ) of MeCP2-deficient cortical PV cells, respectively. The decreased transcription of Kv4.2 , which encodes a fast transient outward K + current ( I A ) channels may count for the increased action potential (AP) half-width in cortical PCs ( Tables 1 and 2 ). These qRT–PCR results for sorted cell populations also suggest a cell-autonomous effect of conditional Mecp2 deletion in PV cells. Table 2 qRT–PCR analysis of the transcription levels of various genes in V1 from PV-Cre;Ai9 control and PV-Mecp2 −/y ;Ai9 mice at P30. Full size table Rescue of OD plasticity by diazepam in PV-Mecp2 −/y mice Taken together, our results from above various experimental assays suggested that selective loss of Mecp2 in PV cells could result in an overall reduction of PV cell-mediated cortical GABA inhibition. This form of inhibition has been known as a critical gate of the onset of critical period for experience-dependent OD plasticity [19] , [22] , [40] . Thus, we further tested whether the reduced level of cortical GABA inhibition potentially accounts for the absence of OD plasticity during the critical period and adulthood of PV-Mecp2 −/y mice. The drug diazepam (DZ), a benzodiazepine agonist of GABA A receptors was used to enhance cortical GABAergic transmission activities with a daily intraventricular infusion for 4–5 days (see Methods). We found that such DZ infusion (2 mg ml −1 , 1.5 μl) 1 day before the 4-d MD, but not the vehicle solution (50% propylene glycol, 49% H 2 O and 1% dimethylsulphoxide), completely restored the MD-induced OD plasticity of the V1 in juvenile PV-Mecp2 −/y mice (P30, Fig. 7a,b ). We also found the same rescuing effect of DZ infusion in the adult PV-Mecp2 −/y mice (P60, Fig. 7c,d ), using relatively higher dose of DZ (4 mg ml −1 , 1.5 μl, due to the increased cortical volume). Previous studies have demonstrated that the minimal 2-day DZ infusion induces the onset of critical period for experience-dependent cortical plasticity primarily through its action on cortical PV cell circuits [22] , [24] , [41] . Thus, these results provide strong evidences for supporting the idea that selective synaptic dysfunctions in local MeCP2-deficient PV cell circuits lead to aberrant experience-dependent cortical plasticity in both juvenile and adult mice. 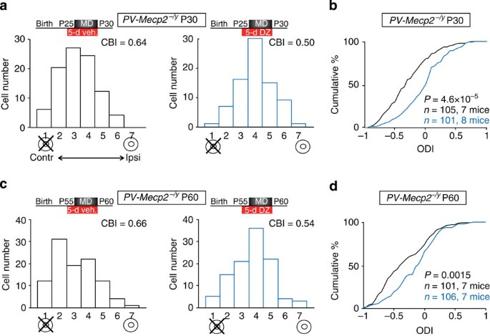Figure 7: Brain infusion of DZ rescues OD plasticity ofPV-Mecp2−/ymice in the critical period and adulthood. (a) 7-Scale histograms of OD of V1 neurons from P30PV-Mecp2−/ymice that were infused with DZ (blue) 1day before MD or the vehicle solution (black). (b) Cumulative percentage distribution of ODI values shown ina. (c,d) 7-Scale histograms and cumulative percentage distribution of ODIs for P60PV-Mecp2−/ymice with DZ (blue) or vehicle (black) infusion before 4-d MD.P-values were calculated by Kolmogorov–Smirnov test. Figure 7: Brain infusion of DZ rescues OD plasticity of PV-Mecp2 −/y mice in the critical period and adulthood. ( a ) 7-Scale histograms of OD of V1 neurons from P30 PV-Mecp2 −/y mice that were infused with DZ (blue) 1day before MD or the vehicle solution (black). ( b ) Cumulative percentage distribution of ODI values shown in a . ( c , d ) 7-Scale histograms and cumulative percentage distribution of ODIs for P60 PV-Mecp2 −/y mice with DZ (blue) or vehicle (black) infusion before 4-d MD. P -values were calculated by Kolmogorov–Smirnov test. Full size image In this study, we show that specific Mecp2 deletion in GABAergic PV cells abolishes the visual experience-dependent OD plasticity during the critical period in postnatal development of V1, while conditional Mecp2 deletion in GABAergic Sst cells or glutamatergic PCs has no such effect. The selective loss of Mecp2 in PV cells causes a substantial reduction of their visual spiking response, but does not affect general visual functions of major V1 excitatory cells. MeCP2-deficient cortical PV cells showed relatively immature membrane properties, selective synaptic deficiency of their afferent excitatory synapse from neighbouring cortical PCs and decreased expression of some related genes, including Gad2 , Parvalbumin , Kv3.1 , Gabra1 , Gabra2 , Calretinin and Glur3 . In contrast, in mice with selective Mecp2 deletion in PV cells, glutamatergic PCs show the unaffected transcription of these examined genes as well as normal membrane excitability and PC-PC synaptic circuits. Overall, these cell-autonomous effects of Mecp2 deletion in PV cells at levels from the molecule to the circuit lead to defective cortical PV cell circuits and absence of experience-dependent critical period OD plasticity in the V1. Thus, our results suggest that MeCP2 expression in GABAergic PV cells in the sensory cortex is essential for maintaining local circuit functions underlying experience-dependent cortical circuit refinement during the postnatal brain development. The expression level of MeCP2 is relatively low at birth but increases greatly within the first 3 weeks of the postnatal development [42] . The latter time course of MeCP2 expression coincides with a postnatal window in which synaptic wiring processes are most active in the brain, and loss-of-function mutations of Mecp2 may lead to disruption of neural circuits [7] . For example, in the dorsal lateral geniculate body, Mecp2-null mice showed normal formation of the retinogeniculate synapses in the early vision-independent phase, but an aberrant remodelling and segregation of these synapses from the two eyes during the late vision-dependent phase [43] . Furthermore, a previous study in Mecp2 heterozygous female ( Mecp2 +/− ) mice showed that OD plasticity was still present in the adult V1 (refs 44 , 45 ). Although the heterozygous mice had significant lower and complex mosaic expression of MeCP2 in neurons due to X-chromosome inactivation, their results imply that the remaining MeCP2 expression in these mice may be still sufficient to maintain the OD plasticity. In the present study, we have provided direct evidence that MeCP2 expression in the inhibitory PV cell circuits is required for experience-dependent refinement of synaptic circuits during the critical period. We also showed that specific loss of Mecp2 in inhibitory Sst-expressing interneuron or excitatory PCs do not impair the critical period OD plasticity. Our findings underscore the notion that PV cell circuit is a critical factor in gating the emergence of critical-period cortical plasticity during the postnatal development [19] , [22] . Previous studies have shown that synaptic function including basal synaptic transmission and plasticity were reduced in mice with constitutive Mecp2 loss ( null ) or specific Mecp2 deletion from GABAergic neurons [7] , [46] . However, most synaptic defects were revealed by recording miniature synaptic events of excitatory or inhibitory transmission [8] , [11] , [18] , [47] , which fails to distinguish inputs from specific neuronal subtypes or circuits. In the present study, our slice recording results directly reveal that the most significant dysfunction of layer 4 PV cells resided in the neighbouring PC’s excitatory input to the PV cell, instead of the PV cell’s inhibitory outputs after the selective loss of Mecp2 in PV cells during critical period ( Fig. 6 ). This selective defect of cortical PC–PV excitatory synapses could directly account for the decrease in the visually evoked spiking rate of MeCP2-deficient cortical PV cells during in vivo recording ( Fig. 4 ), because synaptic strength and excitation/inhibition balance of thalamocortical inputs to the cortical layer 4 were not altered in the PV-Mecp2 −/y mice ( Fig. 6 and Supplementary Fig. 4 ). Moreover, MeCP2-deficient cortical PV cells retained higher input resistance and reduced ability of faithful spiking to high-frequency inputs, presumably caused by decreased expression of Kv3.1 potassium expression ( Table 2 and ref. 48 ), during the critical period and adulthood. However, the higher membrane excitability of MeCP2-deficient PV cells could counter the impact of reduced recurrent excitatory drive onto PV cells, thus retaining an unchanged level of baseline spontaneous spikes of cortical PV cells in the PV-Mecp2 −/y mice in vivo ( Fig. 4 ). All these defects in neuronal and synaptic functions of cortical PV cells are endorsed by the altered transcriptions of related functional genes in MeCP2-deficient cortical PV cells ( Table 2 ). The collective effects from the molecule to the circuit, resulted from Mecp2 -deletion in PV cells, may cause an overall reduction in the level and the fine control of PV cell-mediated recurrent inhibition in the layer 4 local circuits. This could lead to the failure of visual experience-induced synaptic competition underlying OD shift after MD, given the well-known role of PV cell circuits in regulating the critical period [19] , [22] , [40] . In support of the idea, the rescue of OD plasticity in both young and adult PV-Mecp2 −/y mice by DZ infusion was observed. Accumulating evidence has suggested that specific loss of Mecp2 in different neuronal types in various brain areas may contribute to the deficit of a particular behavioural phenotype of RTTs [14] , [15] , [16] , [17] . Our current study demonstrates that the mice with selective deletion of Mecp2 in PV cells in the brain do not recapitulate most RTT-like behavioural phenotypes but similar motor dysfunctions to that observed in RTT patients [2] , [3] . However, we further show an absence of MD-induced OD plasticity in the developing and adult V1 in these conditional KO mice, suggesting a particular role of MeCP2 in specific inhibitory circuits for gating the critical period for experience-dependent modifications of synaptic connections in the sensory cortex. The absence of this form of critical period plasticity in the V1 may lead to impairment in the development of binocularity and the binocular matching of orientation preference in visual cortical cells [49] , [50] . Considering our findings of relatively intact of general RF and tuning properties of V1 cells in these conditional PV-Mecp2 −/y mice ( Figs 1c–h and 3a–d ), we think that the above impairments possibly lead to specific dysfunctions in binocular vision and depth perception in the animal model and RTT patients. It remains to be further examined, as previous studies reported that RTT patients have reduced event-related potentials in electroencephalography recording from sensory cortex [51] , [52] . Similar aberrant critical period plasticity has been found in several other models of the autism spectrum disorder, such as the Fmr1 KO mouse model for fragile X syndrome [53] , [54] and the Ube3a mouse model for Angelman syndrome [55] , [56] . In comparison with mutation in all neurons, deletion of these genes in specific neuronal types may also cause disruption in synaptic remodelling of neural circuits during development. In summary, we demonstrate that during critical period, selective deletion of RTT-related gene Mecp2 in GABAergic PV cells resulted in a defective inhibitory PV cell circuits in developing V1, leading to an absence of experience-dependent critical period plasticity. In general, mutations of these disorder genes in selective neuronal types may also lead to the deficiency in experience-dependent synaptic refinements and neural developmental defects associated with the autism spectrum disorder. Animals Neuronal cell-type-specific deletion of Mecp2 was achieved by crossing different cell-type-specific Cre knock-in lines with heterozygous conditional female mice carrying two functional loxP sites flanking exons 3−4 of Mecp2 on the X chromosome ( flox-Mecp2 or Mecp2 tm1Bird , Jax No.7177) [5] . Only male offsprings were used in the experiments. To specific deletion of Mecp2 in PV-positive GABAergic cells, PV-Mecp2 −/y mice were generated by breeding the offspring of heterozygous female flox-Mecp2 mice to PV-IRES-Cre homozygous male mice (Jax No. : 8069, generated by S Arbor, FMI). Sst-Mecp2 −/y and Nex-Mecp2 −/y mice were obtained by breeding flox-Mecp2 to Sst-IRES-Cre (J.Z. Huang, CSHL; Jax No. 13044) and Nex-Cre lines [57] , respectively, to achieve specific deletion of Mecp2 in Sst-positive GABAergic cells or excitatory glutamatergic neurons. The tdTomato reporter Ai9 mice (Rosa-CAG-LSL-tdTomato-WPRE; Jax No. 7909, generated by H. -k Zeng, Allen Brain Institute, see ref. 26 ) were bred with PV-IRES-Cre or PV-Mecp2 −/y mice to specifically label PV cells with fluorescent proteins (tdTomato). All mice belong to the C57BL/6J strain were reared on a 12/12 h light/dark cycle. The protocols of mouse breeding, care and experimentation were approved by the Animal Care and Use Committees of Shanghai Institutes for Biological Sciences, Chinese Academy of Sciences (Ref. No. NA-100418) and the State Key Laboratory of Cognitive Neuroscience and Learning at Beijing Normal University (IACUC-BNU-NKLCNL-2013-10). Eyelid suture and drug infusion The eyelid suture and drug infusion to the brain were performed to mice of various genotypes and ages under the anaesthesia of isoflurane (1−3% in oxygen, Matrx Vip300 ventilator). The eyelid suture was performed on one eye in mice at desired postnatal stages, for example, P26 or P56, as described previously [21] . The area surrounding the eye was wiped with 70% ethanol. The lid margins were trimmed and then the eye was flushed with saline. Two mattress sutures were placed using the 6-0 silk. After recovery from the anaesthesia, the mice were exposed to normal 12/12 h light/dark rhythm and checked daily to ensure the sutured eye remained closed and uninfected for 4 days. The procedure of daily infusion of DZ to the mouse brain followed a previously described method [40] , [41] , [58] , with some modifications. Mice were anaesthetized with isoflurane and stereotaxically injected with 1.5 μl DZ (2 or 4 mg ml −1 in a vehicle solution containing 50% propylene glycol, 49% H 2 O and 1% dimethylsulphoxide) into the lateral ventricles of both hemispheres (coordinates from Bregma: anteroposterior, −0.3 mm; mediolateral, 1 mm; dorsoventral 2.5 mm), and each side injection was completed within 10 min. The injection was started 1 day before the MD treatment, and made consecutively for 4 days during the MD under the red-lamp lighting. The stereotaxic position of the lateral ventricles for the drug injection was confirmed with fluorescence dye ( Alexa-fluo 488 10-kDa Dextran conjugate, Invitrogen) as in our previous study [40] . Visual stimulation Visual stimuli were generated by custom-developed software using the LabView (National Instrument) and the MatLab (Mathworks), and were presented on a 21-inch cathode ray tube monitor (Sony Multiscan G520, 40.5 × 30.5 cm, refresh rate of 60 Hz, maximum luminance of about 80 cd m −2 ). The cathode ray tube monitor was placed ~20 cm in front of the mouse, subtending about 105° × 80° of the visual field. Two home-customized electromechanical shutters were put close to the eyes and alternatively opened by electric pulses to achieve monocular visual stimulation. All experimental sessions began with full-screen drifting sinusoidal gratings of varying orientations and spatial frequency from 0 to 360° (step at 45°) and 0.001−0.32 cycle per degree (temporal frequency, 2 Hz), respectively, to determine the preferred orientation and spatial frequency of recorded V1 cells. For testing the OD of spiking response of recorded V1 binocular neurons, drifting gratings at the optimal orientation for the contra- and ipsilateral eyes were used, with spatial frequency of 0.02 cycle per degree and temporal frequency of 2 Hz. Each stimulation trial consisted of 1 s of blank screen and 3 s of drifting gratings. In experiments quantifying the OD with extracellular single-unit recordings, full-screen drifting gratings with optimal orientation were used. Each trial consisted of 2 s of drifting gratings and 3−4 s of blank frames. We followed a method of a previous study [59] to map the spatiotemporal RFs of recorded V1 cells on the spike rate. For each neuron, the spatiotemporal RF was estimated by correlating the peristimulus time spike histogram with the bright squares in an 8 × 8 grid. Individual squares (size of 9−11°, full contrast) in the grid were generated in a pseudo-random sequence at a frame rate of 20 Hz. Each position had 50 or 100 repetitions. For two-photon laser imaging guided cell-attached recording, the RF was mapped using a set of flash squares, in which a bright square was flashed in an 8 × 8 grid on a black background. The flash spots were displayed individually in a pseudo-random sequence, with a 120-ms duration and 480 ms interstimulus interval. Each location was stimulated six times. In vivo extracellular or cell-attached recording Mice were anaesthetized by an intraperitoneal injection of ketamine (50 μg g −1 weight)/medetomidine (0.6 μg g −1 ) and mounted on a custom-built mouse stereotaxic device (RWS Life Science, China) during the surgery and recording. The animal heart rate and body temperature were monitored for the state of anaesthesia. Body temperature was maintained at 37 °C by a homeostatically controlled heating pad (RWS Life Science). For extracellular recording, a craniotomy was made over the binocular zone (about 3 mm lateral lambda [21] ) of the mouse V1 in a hemisphere contralateral to the sutured eye [21] , [60] and the dura mater was carefully removed. Eye drops were applied when necessary to prevent the eyes from drying. Single-unit spiking activity was extracellularly recorded with borosilicate glass microelectrodes (Sutter, tip opening 2 μm) and Axon 700B microelectrode amplifier (Molecular Devices). The glass micropipettes were filled with the artificial cerebrospinal fluid (aCSF) containing (in mM) 124 NaCl, 2.5 KCl, 2 MgCl 2 , 2 CaCl 2 , 1.25 NaH 2 PO 4 , 26 NaHCO 3 and 11 D -glucose (pH 7.35, ~303 mOsm), and its resistance was 5–7 MΩ. To quantify the OD distribution of visual cortical cells in the binocular zone, glass micropipettes were penetrated from the superficial to deep cortical layers for 3−4 times and generally 8−12 cortical cells were assayed across the medio−lateral extension of the binocular zone for each mouse. To specifically record from cortical PV cells, in vivo two-photon laser imaging guided cell-attached recording was performed in adult PV-Cre;Ai9 and PV-Mecp2 −/y ;Ai9 mice (P60–65). In this set of experiments, visual stimuli were presented to the contralateral eye through a LCD monitor (7 inch, Xenarc Technologies Corp.; refresh rate 75 Hz) at a distance of 10 cm away. Under the same ketamine/medetomidine anaesthesia, a cranial window of 2 × 2 mm was made over the V1 for two-photon imaging and a glass coverslip was attached to the craniotomy using dental cement around its edges. The aCSF solution containing Alexa Flour 488 (50 μM, Molecular Probes) was added into glass micropipettes (with tip opening of ~2 μm and 6–10 MΩ resistance) to visualize the pipette tips during the imaging. The micropipette was advanced to the pia at a 14° angle with a micromanipulator (Sutter, MP-255). After contacting the pia, the pipette was advanced at the step of 1 μm toward tdTomato-expressing cells within V1 layer 2/3 under the guidance of continuous two-photon imaging. The 960-nm two-photon laser was used to excite Alexa 488 and tdTomato fluorescence. During the procedure of pipette advancing in the cortical tissue, a pressure of 0.2 psi was applied to the micropipette until the pipette touched the cell membrane, indicated by large drop in the magnitudes of currents responding to testing voltage pulse (5 mV, 100 Hz). The positive pressure was then released and a small amount of suction was immediately applied to form loose seal of resistances ranging from 30 to 800 ΩM. This loose-seal configuration recorded spikes from a single cell without rupturing cell membranes. Extracellular or membrane voltage changes were recorded with an Axon MultiClamp 700B (Molecular Devices). Electric signals were filtered at 5 KHz (low pass), digitalized by a Digidata 1440A converter board (Molecular Devices) and acquired at 10 KHz with the pClamp10 (Molecular Devices) into a computer for further analysis. Spikes were detected and sorted off-line using the Offline Sorter (Plexon Inc,) and further analysed by a custom programme in the MatLab (Mathworks). The baseline spike activity was defined by the average spike number within 1 s before the onset of grating stimuli. Spikes evoked by visual stimuli were counted over the duration of visual stimulation (for example, 3 s for drifting gratings) and average rates were presented as spikes per second, after the subtraction from the average baseline activity. Cortical slice preparation and in vitro electrophysiology The preparation of visual cortical slices from young (P28−P30) and adult (P50) male WT, flox-Mecp2 , PV-Cre;Ai9 (control) or PV-Mecp2 −/y ;Ai9 mice and whole-cell recording from V1 layer 4 neurons followed a method described in our previous studies [34] , [35] . The different genotype mice at designed postnatal ages were anaesthetized with sodium pentobarbital (50 μg g −1 ) and decapitated. The brain was rapidly dissected and transferred into ice-cold aCSF (saturated by 95% O 2 ) for 2 min. Coronal slices (350- to 400-μm-thick) of the neocortex were prepared with Vibratome (St Louis, MO) at 0–2 °C to prepare visual cortical slices and further incubated with oxygenated aCSF at 34 °C for 30 min. The cortical slices were then transferred to aCSF at room temperature (25 °C) for >30 min before use. For recording experiments, visual cortical slices were transferred to the recording chamber and perfused with oxygenated aCSF (~2 ml min −1 ) at 31–33 °C (TC-324B, Warner). Whole-cell recording from layer 4 PV and PCs in slices was performed with an Axon 700B amplifier (Molecular Devices). The internal solution contained (in mM): 130 K-gluconate, 20 KCl, 20 HEPES, 0.2 EGTA, 4 ATP-Mg, 0.3 GTP-Na and 10 phosphocreatine-Na (pH, 7.2, ~298 mOsm), and the resistance of glass micropipettes was 3–4 MΩ. In some recording experiments, biocytin (0.2%) was included in the internal solution for neuronal morphology reconstruction. The membrane properties and spiking ability of recorded cells were assayed by intracellular injection of step currents (600 ms duration, magnitudes ranging up to 1 nA with steps of 40–50 pA). To assay the efficacy and short-term plasticity of synapses between paired PC and PV cells or paired PC and PC, a train of five pulses (1 ms duration at 20 Hz) was applied to the presynaptic neuron (in the current-clamp) at a low frequency of 0.033 Hz. Evoked monosynaptic EPSCs or IPSCs were recorded in postsynaptic neuron in the voltage clamp ( V clamp =−70 and −40 mV, respectively). One single spike was elicited 0.5 s after the train stimulation to measure the synaptic recovery rate. In the experiments of assaying distal projection inputs, same pattern train stimulation was delivered through a concentric tungsten electrode (125 μm outer diameter) to the cortical white matter area, at the minimal stimulation intensity that evoked excitatory transmission with a failure rate of 30–40%. The evoked EPSCs of projection synapses were recorded in the presence ( Fig. 6c,d ) or absence ( Supplementary Fig. 4a,b ) of PTX (20 μM). For obtaining the evoked inhibitory and excitatory conductances in layer 4 PCs, IPSCs and EPSCs were recorded from a layer 4 PC at the membrane potentials of 0 mV and −85 mV (after the calibration of pipette junction potentials) in the voltage-clamp configuration in the absence of PTX in the aCSF, respectively, following the electric stimuli at three increasing intensities above the minimal intensity via a concentric tungsten electrode. In the experiment of recording Na + or K + current, the activated sodium current was isolated at voltage clamp in the presence of the blockers for K + channels tetraethylammonium (20 mM) and 4-aminopyridine (3 mM), as well as the blocker for Ca 2+ channels CdCl 2 (0.1 mM). The K + current was recorded in the presence of CdCl (0.1 mM) and tetrodotoxin (500 nM). Electric signals were filtered at 5 KHz (low pass), digitized (Digidata 1322A, Molecular Devices) at 10 (for synaptic events) or 100 KHz (for action potentials) with the pClamp 10 (Molecular Devices) into a computer for further analysis. Data were accepted for analysis only for recording cases in which the magnitude of serial resistance varied <20% throughout the experiments. Immunohistochemistry and confocal imaging Mice were fixed by transcardial perfusion with 4% paraformaldehyde after in vivo recording. Dissected brains were removed and fixed with paraformaldehyde at 4 °C, and cryoprotected with 30% sucrose and then cut into 30 μm coronal sections on a Leica HM525 cryostat. Cortical sections were incubated with rabbit polyclonal antibody against MeCP2 (1:1,000, Cell Signaling Technology), goat polyclonal antibody against somatostatin (1:1,000, Santa Cruz Biotechnology), rabbit polyclonal antibody against GABA (1:1,000, Sigma-Aldrich), mouse monoclonal antibody against PV (1:1,000, Millipore) and NeuN (1:500, Millipore) overnight at 4 °C. Secondary antibodies, Alexa Fluor 488 donkey against rabbit IgG antibody (1:1,000, Invitrogen) and Alexa Fluor 568 antibody against mouse IgG antibody (1:1,000) were used. The nuclei were stained with DAPI (4′,6-diamidino-2- phenylindole). Fluorescence images of the V1 sections were acquired using a Nikon A1 confocal microscope with × 20 or × 60 oil emersion objective lens, using z -stacks at 1 μm steps. In the experiments measuring the PV axonal density in the V1, PV- Cre;Ai9 and PV-Mecp2 −/y ;Ai9 mice were processed simultaneously. For qualification of PV cell axon puncta (tdTomato) on the soma of layer 4 PCs (NeuN staining), maximum intensity projection of z -stack images were acquired. The images of the peri-somatic area of PCs were then cropped from each stack to reconstruct three-dimensional morphology and quantified by the total puncta volume and number enwrapping the PC soma and the bordering space 2 μm away from soma membrane, using NIH Image J software. Both tdTomato and NeuN staining fluorescence signals were processed by setting a constant threshold to eliminate background. Only the tdTomato (PV cell axon) puncta with at least 1 voxel overlap with the PC soma (NeuN staining) were taken as axonal puncta contacting the PC soma. The puncta density was defined as the ratio of the total puncta number and PC soma surface area. FACS and qRT–PCR analysis Transgenic mice at P30−35 were deeply anaesthetized with isoflurane, the visual cortices were dissected in a chilled Earls balanced salt solution. The tissue was dissociated for 40 min at 37° with Papain enzyme (Papain Dissociation System, Worthington Biochem) and then triturated to obtain cells. The cell suspension was centrifuged at 900 r.p.m. at room temperature for 5 min. To remove the debris, cell pellets were re-suspended in Earls balanced salt solution, DNase and albumin ovomucoid inhibitor and the suspension was centrifuged on an albumin ovomucoid inhibitor gradient at 1,000 r.p.m. for 5 min. Cells were treated with propidium iodide (5 μg ml −1 ) to label dead cells and sorted on Beckman Coulter MoFlo XDP. WT non-fluorescent neurons were used to set the side and forward scatter. The single fluorescence-labelled samples were used to set the sorting gate. The test samples were finally analysed and sorted. Both the fluorescent and non-fluorescent cells were collected for further analysis. For qRT–PCR assays, total RNA was extracted from mouse cortical tissues using mirVana miRNA Isolation Kit (Ambion). Complementary DNA was synthesized from 500 ng of purified RNA by iScript cDNA Synthesis Kit (BioRad). SYBR Premix Ex Taq from Takara was used. qRT–PCR was performed with the Rotor-Gene Q machine (Qiagen). Results were normalized to glyceraldehydes 3-phosphate dehydrogenase and data analysis was done by using the comparative C T method in software by Qiagen. The detail of primers was shown in the Supplementary Table 1 . Behavioural tests The mice were first evaluated for general health including appearance of the fur and body weight. All behavioural studies began 1 week after moving to the animal facility. The mice were habituated to the testing room for ~30 min before the test. WT, PV-Cre , flox-Mecp2 and PV-Mecp2 −/y mice at 8~10 weeks of age were used for all behavioural assays. All of the genotypes were blind when behavioural tests were carried out. The number of mice was noted in the legend. Data are shown as mean±s.e.m. and analysed by one-way analysis of variance with Tukey’s post hoc analysis. Accelerating rotarod test . This assay was used for testing locomotor balance and coordination [61] . The mice were placed on an accelerating, 3-cm-diameter rotarod for 12 trials (4 trials per day for 3 days). Each trial was set at an initial value of 4, with linearly increasing to a maximum of 40 r.p.m. across the 5-min test. Latency to fall was recorded by the rotarod timer. The mean latency to fall over the two trials was the reliable. Data were analysed with repeated measures two-way analysis of variances with Bonferroni’s post hoc analysis. Three-chamber test . The social interaction test was performed as previously described [18] , [61] with some modifications. The three-chamber apparatus is a rectangular plexiglass box (60 × 40 × 30 cm) with partitions evenly divided into left, centre and right chambers. Ambient light was 12 lux and background noise was maintained at 60 dB. (A) Habituation: During the habituation period, the test mouse was placed in the middle chamber and allowed to explore for 15 min. Each side contained an empty wire cage with a plexiglass box on top of the cage to prevent climbing by the test mice. The measures were taken of the total time the test mouse spent in each side. (B) Sociability: The age-matched C57BL/6 stranger mice (adult males) were housed in separated cages and habituated to the wire cages for 1 h at 2 days before the social testing. The location of the novel mouse was placed randomly between the right and left chambers. The empty wire cage served as an inanimate object and as a container control for novel mouse. The test mouse was placed in the centre chamber and allowed to explore the entire apparatus for 15 min. Measurements were recorded for the amount of time spent in each chamber and the amount of time spent sniffing, pawing at each wire cage using a video tracking system and EthoVision software (Noldus Information Technologies). Open-field test . Exploratory locomotor activity was measured in an open field (40 × 40 × 40 cm) [61] . Overhead lighting was maintained at 12 lux and background noise was 60 dB. Mice were placed in the centre and allowed to explore freely in 30-min period. The total distance, the centre distance and the entries to the centre were recorded and tracked with EthoVision software (Noldus Information Technologies). Elevated plus maze . The plus maze, which is elevated 50 cm above the floor, comprised two open arms (30 × 15 × 5 cm) and two closed arms (30 × 15 × 5 cm) across from each other. Mice were placed in the centre section facing the open arm and allowed to explore for 5 min. Global activity was assessed by the number of visits and duration in the open and closed arms with observer programme (Noldus Information Technologies). Light–dark box . The light–dark box consisted of a clear plexiglass chamber (light side, 30 × 30 × 27 cm) and a covered black chamber (dark side, 30 × 27 × 15 cm) separated by a blank partition with a small opening. The lighting maintained at 700 lux and the white noise was 60 dB. The mouse was placed into the dark compartment and allowed to explore for 10 min. Measurements were taken of the number and latency of entries, and the time and distance in each side. Fear-conditioning test . The fear-conditioning protocol was designed as previously described with modification [62] . Mice were placed in individual chambers for 2 min followed by a 5-KHz pure tone (90 dB, 30 s duration) and a 0.5-mA foot-shock for 2 s. Three rounds of training were performed with variable intervals. Contextual memory was tested 24 h later by placing mice back in the same boxes without a tone or shock. The cued memory was performed by placing mice in a novel context without shock or sound for 3 min, followed by 3 min of the tone stimuli. The total amount of time spent in freezing was recorded. Data analysis The OD preference of each recorded cell in the V1 binocular zone was defined by an OD index (ODI) as: where R ipsi and R contra represent the average spike rates evoked by the visual stimuli presented to the contra- and ipsilateral eyes, respectively, after the subtraction of baseline spiking rate. The index ranges from +1 for neurons driven exclusively by the ipsilateral eye to −1 for those driven exclusively by the contralateral eye. Cells were assigned OD scores according to the classical 7-point scale, and then the CBI was calculated as: where N was the total number of cells and n x were the number of cells with an OD score equals to x in the 7-point scale [21] , [63] . The strength of orientation selectivity was quantified with a global measure of orientation selectivity [30] , [64] , [65] , [66] : where θ i is the angle of the moving direction of the grating. R ( θ i ) is the spike response amplitude (with baseline subtracted) at angle θ. The conductance of Na + and K + were determined as: where I is the peak current at each test pulse, E Na is the reversal potential of Na + currents (+55 mV), while E K is the reversal potential of K + currents (−90 mV). The conductance–voltage activation curve was fitted by the Boltzmann equation: where G was the membrane conductance at potential V , V 1/2 was the half activation and k was a slope factor. Data are presented as mean±s.e.m. unless stated otherwise. The statistical significance was tested with the two tail t -test when the data were in the normal distribution. For data with non-normal distributions, statistical significance was tested with non-parametric Mann–Whitney test instead. For testing the significance of the difference in the distributions of ODI or synaptic current amplitude, Kolmogorov–Smirnov test was used. How to cite this article: He, L.-j. et al . Conditional deletion of Mecp2 in parvalbumin-expressing GABAergic cells results in the absence of critical period plasticity. Nat. Commun. 5:5036 doi: 10.1038/ncomms6036 (2014).